Lipid tail protrusions mediate the insertion of nanoparticles into model cell membranes Recent work has demonstrated that charged gold nanoparticles (AuNPs) protected by an amphiphilic organic monolayer can spontaneously insert into the core of lipid bilayers to minimize the exposure of hydrophobic surface area to water. However, the kinetic pathway to reach the thermodynamically stable transmembrane configuration is unknown. Here, we use unbiased atomistic simulations to show the pathway by which AuNPs spontaneously insert into bilayers and confirm the results experimentally on supported lipid bilayers. The critical step during this process is hydrophobic–hydrophobic contact between the core of the bilayer and the monolayer of the AuNP that requires the stochastic protrusion of an aliphatic lipid tail into solution. This last phenomenon is enhanced in the presence of high bilayer curvature and closely resembles the putative pre-stalk transition state for vesicle fusion. To the best of our knowledge, this work provides the first demonstration of vesicle fusion-like behaviour in an amphiphilic nanoparticle system. Nanomaterials are used in nanomedicine with applications ranging from drug delivery [1] , [2] , [3] to biosensing [4] and bioimaging [5] , with several companies already utilizing such platforms in advanced clinical trials. However, their potential as therapeutic agents largely depends on the ability to precisely control their fate once inside the body to achieve the desired effect without adverse consequences. In order to resolve this challenge, it is essential to understand the interactions between nanomaterials and the cellular machinery. Gold nanoparticles (AuNPs) offer an ideal platform for exploring the interactions between nanomaterials and the cell membrane [6] ; their size can be controlled [7] and their surface properties can be finely tuned by grafting a protecting ligand monolayer [8] , [9] , [10] that provides stability and control over surface structure and composition. Grafting a monolayer of alkanethiol ligands with different end groups is particularly suitable for biological applications, since it is possible to mimic the surface properties of a typical globular protein in terms of chemistry, size and solubility. For example, the combination of hydrophobic alkane backbones and hydrophilic end groups can yield amphiphilic surface properties [9] , [11] . Such amphiphilicity has already been proven to be an important factor in determining the interactions between biological nanoobjects, such as cell-penetrating peptides, and either the cell membrane or a lipid bilayer [12] , [13] , [14] . Similar interactions between monolayer-protected AuNPs and lipid bilayers have been a subject of intense investigation by experimental and theoretical studies aimed at eliciting the role of surface charge, ligand composition and particle size among other tuning parameters on nano–bio interactions [6] , [15] , [16] , [17] , [18] , [19] , [20] , [21] , [22] , [23] . Recently, using both experiments and free-energy calculations, we showed that water-soluble, amphiphilic AuNPs protected with a binary mixture of alkanethiol ligands were able to insert into and fuse with the hydrophobic core of lipid vesicles and suspended lipid bilayers [24] , [25] . The amphiphilic properties of the AuNPs resulted from the combination of the hydrophobic alkane backbones and the presence of a variable percentage of anionic sulphonate end groups [9] . We demonstrated that this fusion process was regulated by the size of the AuNP with a composition-dependent size threshold [24] , [25] . In particular, AuNPs with core diameters smaller than ~3.0 nm fused independent of monolayer composition or surface structure [25] . Moreover, the same AuNPs that inserted into lipid vesicles were also observed to spontaneously penetrate into cells if their core diameters were below the same size threshold, indicating the importance of bilayer fusion as a precursor to cell entry [25] , [26] , [27] . The thermodynamic driving force for insertion was the hydrophobic effect: the amphiphilic particle surfaces could eliminate water-exposed hydrophobic surface area by inserting into the hydrophobic bilayer core while retaining hydrophilic end groups in aqueous solution by ‘snorkelling’ [28] , [29] . Other experimental systems have found such complexation as well [30] , [31] . Although these previous studies have elucidated the thermodynamics of nanoparticle insertion into lipid bilayers [24] , [25] , [32] , the detailed kinetics of the insertion process are still unclear. In the present work, we use a combination of atomistic molecular dynamics simulations and experiments to gain insight into the kinetic barriers that may affect the insertion of amphiphilic AuNPs into bilayers. This process must involve the contact between hydrophobic material in the monolayer and the hydrophobic core of the bilayer as in similar situations reported in the literature: for example, recent studies on peripheral protein binding have suggested that hydrophobic residues may contact the hydrophobic core of the bilayer through ‘hydrophobic defects’ [33] , while the pathway of vesicle–vesicle fusion involves the contact of lipid tails via stochastic protrusions into solvent [34] , [35] , [36] , [37] , [38] . Both of these processes are enhanced by bilayer curvature [38] , [39] , [40] . We thus hypothesize that AuNP insertion will be similarly enhanced when AuNPs encounter highly curved bilayers. Unbiased simulations support this hypothesis by showing spontaneous insertion within nanoseconds at the highly curved edge of a bilayer ribbon but not through its planar face. We confirm this result experimentally by showing that AuNPs will enter supported lipid bilayers (SLBs) only in the presence of large defects, and that insertion is localized near defect edges. Having established this agreement between simulations and experiments, we use committor analysis to identify the transition state for AuNP insertion from multiple unbiased trajectories [41] , [42] , and we show that it involves the protrusion of a lipid tail into solvent, a configuration resembling the point-like pre-stalk transition for vesicle–vesicle fusion [43] . To the best of our knowledge, this work provides the first demonstration of vesicle fusion-like behaviour in an amphiphilic nanoparticle system. The use of two opposite extremes of bilayer curvature indicates that significant kinetic barriers may inhibit insertion even when fusion is thermodynamically favourable in low curvature systems, and suggests that these kinetic barriers may be minimized in fusogenic systems. Using unbiased atomistic simulation methods that accurately capture the physicochemical forces acting at this nano–bio interface, we thus demonstrate a lipid tail protrusion-mediated pathway for the spontaneous fusion of soluble charged AuNPs with a bilayer. Unbiased simulations of AuNP-bilayer ribbon interactions We performed unbiased atomistic molecular dynamics simulations to investigate the kinetic pathway of AuNP insertion into lipid bilayers. As a model system, we simulated small, amphiphilic monolayer-protected AuNPs with core diameters of 2.0 nm. The simulations of the AuNP-bilayer interactions were performed using a recent parameterization of mixed monolayer-protected AuNPs [44] . The simulations use the GROMOS 54a7 force field that is parameterized from free energies of solvation [45] , [46] and has been recently shown to accurately reproduce bilayer structural properties [47] . Unless otherwise noted, each AuNP had a diameter of 2.0 nm and surface grafting density of 4.62 ligands per nm 2 , leading to 58 ligands per particle in agreement with previous studies [48] . To mimic previous experimental systems, the surface monolayer was either all-MUS (11-mercapto-1-undecanesulphonate) or a mixture of MUS with OT (1-octanethiol) in a stoichiometric ratio of 1:1 MUS:OT [24] , [25] , [26] , [27] . MUS has an alkane backbone and a hydrophilic anionic sulphonate group, whereas OT is purely hydrophobic ( Fig. 1 ). These two compositions were chosen such that AuNPs with intermediate compositions would likely exhibit behaviour either similar to or lying between the two extremes. In principle, the organization of the two ligand species in the 1:1 MUS:OT monolayer could influence properties; for example, the arrangement of ligands into an alternating stripe-like pattern was shown to enhance cell penetration [26] , [27] . However, recent work indicated that surface structure does not significantly affect the proposenity for small AuNPs to fuse with single component bilayers [25] , and furthermore small AuNPs exhibit similar structural characteristics in water independent of morphology [44] . Experimental evidence also suggests that for small AuNPs, the two ligand species fully separate to form Janus particles [49] . However, the expected electrostatic attraction between the MUS end groups and the bilayer would cause the MUS ligands in the Janus morphology to approach the surface in the same orientation as for an all-MUS particle [20] . Comparing the behaviour of all-MUS and MUS:OT AuNPs is thus sufficient to explore the effects of the amphiphilic character of the surface composition independent of the surface structure of the monolayer. Additional details of the AuNP parameterization are found in the Supplementary Methods . 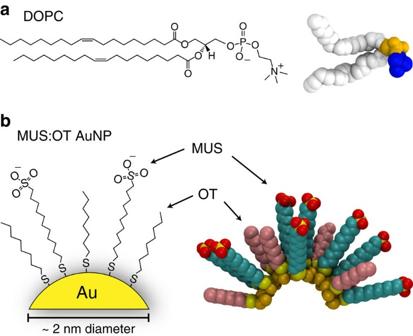Figure 1: Summary of system components used for both simulations and experiments. (a) Chemical structure and simulation snapshot of the zwitterionic lipid DOPC used to create the bilayers. The gel–fluid transition of the bilayer occurs atTm=−21 °C, well below simulation and experimental temperatures. (b) Chemical structure and simulation snapshot of a MUS:OT AuNP. MUS has a hydrophobic alkane backbone and anionic end group, whereas OT is purely hydrophobic. All experiments and simulations were performed in a physiological 150 mM NaCl salt concentration (not illustrated). Simulation snapshots are rendered using visual molecular dynamics (VMD)70. Figure 1: Summary of system components used for both simulations and experiments. ( a ) Chemical structure and simulation snapshot of the zwitterionic lipid DOPC used to create the bilayers. The gel–fluid transition of the bilayer occurs at T m =−21 °C, well below simulation and experimental temperatures. ( b ) Chemical structure and simulation snapshot of a MUS:OT AuNP. MUS has a hydrophobic alkane backbone and anionic end group, whereas OT is purely hydrophobic. All experiments and simulations were performed in a physiological 150 mM NaCl salt concentration (not illustrated). Simulation snapshots are rendered using visual molecular dynamics (VMD) [70] . Full size image The lipid bilayer was modelled as a DOPC (1,2-dioleoyl-sn-glycero-3-phosphocholine) ‘ribbon’ immersed in a 150-mM NaCl solution with two edges of the bilayer exposed to solvent. The ribbon geometry was assembled by creating a bilayer that is periodic along the y dimension of the simulation box but has water separating the two bilayer edges along the x axis ( Fig. 2 ). At equilibrium, lipids along the two water-exposed edges deform to minimize exposure of the hydrophobic core to water, creating a highly strained edge with extreme curvature. Two possible starting configurations for AuNPs were tested: the AuNP was placed either above the middle of the ribbon ( Fig. 2a,b ) or near the bilayer edge ( Fig. 2c,d ). These configurations are representative of experiments with an AuNP approaching a planar bilayer or highly curved bilayer, respectively. 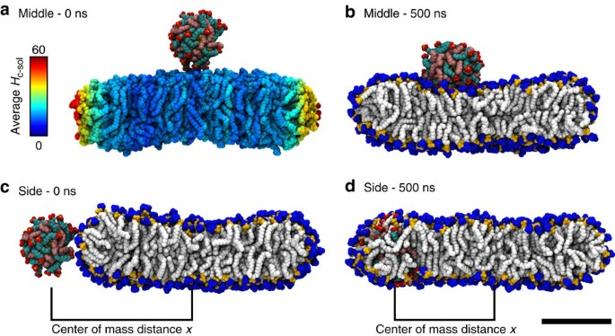Figure 2: Simulation snapshots of interactions between AuNPs and bilayer ribbons. (a) A 1:1 MUS:OT AuNP placed in the middle configuration representative of interactions between AuNPs and planar bilayers. Lipids are coloured byHc-sol, the number of atoms in water molecules that are in contact with hydrophobic lipid tail atoms. Lipids in the planar face have relatively low amounts of water-tail atom contact (dark blue) compared with the much greater tendency of water-hydrophobic tail contact with lipids near the edge (yellow–red). (b) AuNP in the middle configuration after 500 ns. No fusion was observed as the particle only diffuses along the surface (Supplementary Discussion). (c) An AuNP in the side configuration representative of interactions between AuNPs and highly curved bilayers. (d) AuNP in the side configuration after 500 ns. Multiple simulations showed spontaneous insertion for AuNPs from this starting configuration. Scale bar, 5 nm (for all images). Figure 2a further illustrates the distinction between these two starting points by colouring all lipid head groups according to the average number of atoms in water molecules within 0.5 nm of any hydrophobic lipid tail bead, H c-sol . From this image (with corresponding plot in Supplementary Fig. 1 ), it is clear that AuNPs placed near the bilayer edge will encounter lipids that are much more prone to water contact than lipids near the planar face of the ribbon. Figure 2: Simulation snapshots of interactions between AuNPs and bilayer ribbons. ( a ) A 1:1 MUS:OT AuNP placed in the middle configuration representative of interactions between AuNPs and planar bilayers. Lipids are coloured by H c-sol , the number of atoms in water molecules that are in contact with hydrophobic lipid tail atoms. Lipids in the planar face have relatively low amounts of water-tail atom contact (dark blue) compared with the much greater tendency of water-hydrophobic tail contact with lipids near the edge (yellow–red). ( b ) AuNP in the middle configuration after 500 ns. No fusion was observed as the particle only diffuses along the surface ( Supplementary Discussion ). ( c ) An AuNP in the side configuration representative of interactions between AuNPs and highly curved bilayers. ( d ) AuNP in the side configuration after 500 ns. Multiple simulations showed spontaneous insertion for AuNPs from this starting configuration. Scale bar, 5 nm (for all images). Full size image A series of six unbiased 40-ns simulations with a 1:1 MUS:OT AuNP placed in the ‘middle’ configuration showed no insertion, although electrostatic interactions between the anionic MUS end groups and the bilayer attracted the AuNP to the surface. Prolonging one of these simulations to 500 ns showed that the MUS:OT AuNP diffused along the bilayer surface without inserting ( Fig. 2b ). Six similar 40-ns simulations were carried out for both all-MUS and MUS:OT AuNPs placed in the ‘side’ configuration. Three of the six simulations with a MUS:OT particle and one of the six simulations with an all-MUS particle showed spontaneous AuNP insertion into the bilayer. One of the simulations showing insertion for each particle type was prolonged to 500 ns to obtain a full unbiased pathway for spontaneous fusion as shown in Figs 2d and 3 . Simulations with larger 3.0 nm 1:1 MUS:OT AuNPs confirmed that insertion was not restricted to the smaller AuNPs ( Supplementary Fig. 2 ). To gain insight into the insertion pathway, we tracked the evolution of the distance Δ x between the centre of the AuNP and the centre of mass of the ribbon relative to the initial AuNP starting position. Results from the first 100 ns of the 500-ns trajectories are presented in Fig. 3 for both types of AuNP together with snapshots of representative system configurations. Δ x is negative in all cases, consistent with a decrease in the distance between the AuNP centre and ribbon centre from the initial starting position where Δ x =0. 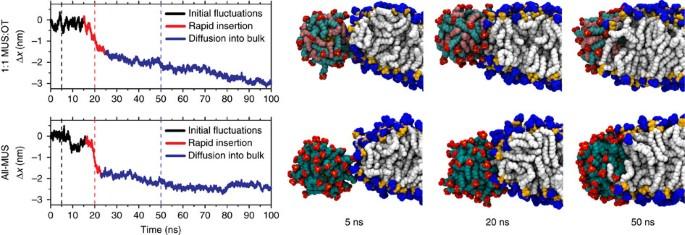Figure 3: Summary of unbiased insertion of both AuNPs. Plots of the change in distance Δxbetween the centre of the AuNP and centre of mass of the bilayer are shown as a function of time for the first 100 ns of insertion for both 1:1 MUS:OT and all-MUS AuNPs.xis indicated inFig. 2. Three regimes of behaviour are indicated by different coloured lines. Representative snapshots corresponding to the times indicated by dashed vertical lines are shown on the right. A plot of Δxfor the full 500 ns is shown inSupplementary Fig. 3. Additional snapshots with either the AuNP or lipid tails removed are shown inSupplementary Fig. 4to clarify the behaviour of hydrophilic and hydrophobic ligands during the insertion. Water and ions are removed for clarity. Figure 3: Summary of unbiased insertion of both AuNPs. Plots of the change in distance Δ x between the centre of the AuNP and centre of mass of the bilayer are shown as a function of time for the first 100 ns of insertion for both 1:1 MUS:OT and all-MUS AuNPs. x is indicated in Fig. 2 . Three regimes of behaviour are indicated by different coloured lines. Representative snapshots corresponding to the times indicated by dashed vertical lines are shown on the right. A plot of Δ x for the full 500 ns is shown in Supplementary Fig. 3 . Additional snapshots with either the AuNP or lipid tails removed are shown in Supplementary Fig. 4 to clarify the behaviour of hydrophilic and hydrophobic ligands during the insertion. Water and ions are removed for clarity. Full size image The insertion of the AuNPs into the bilayer occurred in three stages ( Fig. 3 ). At the beginning of the simulation (black line), the particle first fluctuated through the water surrounding the bilayer, with electrostatic interactions attracting it to the bilayer edge as shown in the first snapshot. A few nanoseconds later, the AuNP rapidly inserted into the bilayer through the highly strained edge as shown by the sharp decrease in Δ x (red line). During this rapid penetration, the hydrophilic end groups were consistently solvated by snorkelling towards the nearest aqueous interface while the hydrophobic ligands of the MUS:OT particle extended into the middle of the bilayer where the density of lipid tail groups was lower. After this period, the AuNP continued to slowly insert into the bilayer until Δ x began to plateau (blue line). In this plateau region, the hydrophilic end groups lined the bilayer edge in a conformation nearly identical to the edge lipids. The trajectories in Supplementary Fig. 3 show that the plateau is reached at smaller Δ x for the all-MUS particle than the MUS:OT particle, likely owing to the lower amount of hydrophobic material in the monolayer. Final configurations after 500 ns are shown in Fig. 2 with additional snapshots in Supplementary Fig. 4 . The unbiased simulations show that both all-MUS and 1:1 MUS:OT AuNPs can spontaneously insert through the highly curved bilayer edge on short simulation timescales, whereas no insertion is observed through the planar bilayer surface. It must be emphasized that these simulations were completely unbiased; no external potential was applied to force AuNP insertion, a technique frequently used in similar simulations [22] , [23] that may induce unphysical system configurations. Experimental results on AuNP–lipid bilayer interactions Using atomic force microscopy (AFM) in liquid and quartz crystal microbalance with dissipation (QCM-D), we were able to monitor and detect in solution the interactions of amphiphilic AuNPs with supported planar lipid bilayers. The SLBs were prepared by fusion of pure DOPC vesicles on a silicon wafer in a standard phosphate (phosphate-buffered saline, PBS) solution and kept immersed in solution for the duration of all the experiments. It was possible to obtain both defect-free SLBs and defect-rich SLBs ( Supplementary Methods ). AuNPs were then added to the PBS solution and incubated with the supported bilayer. We used polydisperse AuNPs with a mean gold core size of 5–6 nm coated with a 2:1 MUS:OT monolayer [24] , [25] , [26] , [27] as an intermediate composition between the all-MUS and 1:1 MUS:OT compositions studied in simulations. These AuNPs were large enough to not form Janus morphologies [49] but sufficiently small that insertion would be expected [25] , [32] . Details of particle characterization are in the Supplementary Methods . An example of a SLB that appears defect free in the area imaged by the AFM is presented in Fig. 4a . The image in Fig. 4b was recorded after the addition of a concentrated 2:1 MUS:OT AuNP solution to obtain a final concentration of approximately 1 mg ml −1 (see Supplementary Fig. 5 for detailed characterization). No substantial changes in the surface topography are observed, suggesting no local interaction between AuNPs and the SLB. Since AFM can only study a small portion of the bilayer surface, we used QCM-D to confirm the uptake of AuNPs by the whole sample [50] , [51] . QCM-D measurements on the perfectly formed bilayer (insets of Fig. 4a,b ) confirmed that no change to the bilayer had occurred upon the addition of AuNPs as evident in the quasi-constant frequency and dissipation signals. For further information see Supplementary Methods . 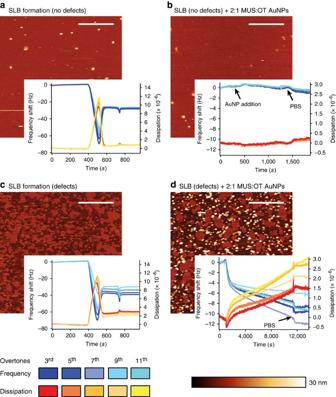Figure 4: 2:1 MUS:OT AuNP interactions with planar SLBs. Interactions are measured with both AFM (images) and QCM-D (insets). (a) Defect-free SLB after formation by vesicle fusion. (b) Defect-free SLB after subsequent addition of a solution of 1 mg ml−12:1 MUS:OT AuNPs in PBS. No evidence of AuNP insertion is observed, as confirmed by QCM-D. Black arrows indicate the times when AuNPs were added and when PBS was added to remove excess particles. (c) Defect-rich SLB after formation by vesicle fusion. (d) Defect-rich SLB after addition of 2:1 MUS:OT AuNPs in PBS. The AFM image indicates that 2:1 MUS:OT AuNPs are now able to interact at defect edges. This finding is confirmed by the large variations in frequency shifts and dissipation in the QCM-D signals. Scale bars, 3 μm (in all AFM images). Figure 4: 2:1 MUS:OT AuNP interactions with planar SLBs. Interactions are measured with both AFM (images) and QCM-D (insets). ( a ) Defect-free SLB after formation by vesicle fusion. ( b ) Defect-free SLB after subsequent addition of a solution of 1 mg ml −1 2:1 MUS:OT AuNPs in PBS. No evidence of AuNP insertion is observed, as confirmed by QCM-D. Black arrows indicate the times when AuNPs were added and when PBS was added to remove excess particles. ( c ) Defect-rich SLB after formation by vesicle fusion. ( d ) Defect-rich SLB after addition of 2:1 MUS:OT AuNPs in PBS. The AFM image indicates that 2:1 MUS:OT AuNPs are now able to interact at defect edges. This finding is confirmed by the large variations in frequency shifts and dissipation in the QCM-D signals. Scale bars, 3 μm (in all AFM images). Full size image Using the same preparation method, but on a different sample, we were able to obtain the bilayer shown in Fig. 4c . It consists of many lipid islands rich in boundaries and separated by distances much larger than the size of the AuNPs. Upon addition of the same MUS:OT AuNPs used for the experiment in Fig. 4b , clear deposition of the particles near and at the SLB boundaries was observed from changes to the bilayer topography. We interpret the localized increase in height as clusters of AuNPs inserting into the lipid bilayer. The QCM-D results substantially confirm this observation. The signals recorded during the SLB formation are presented in the inset of Fig. 4c : the lower value of the QCM-D frequency shift, the split of the overtones and a higher dissipation value are indications of an incompletely formed lipid bilayer. Upon the addition of AuNPs to the defect-rich bilayer ( Fig. 4d ), a decrease in the frequency shift and increase in the dissipation were recorded. This is a clear signature of extra-mass attachment on the sensor. The shifts in frequency and dissipation were maintained even after the removal of extra particles by flowing PBS into the QCM-D chamber (black arrow in Fig. 4d ). Control experiments confirmed that the AuNPs do not adsorb to the bare silicon wafer substrate, further indicating preferential bilayer interactions ( Supplementary Fig. 6 ). The combined AFM and QCM-D data show that MUS:OT AuNP insertion occurs mainly in the presence of membrane defects. To gain an improved understanding of the dynamics and spatial localization of the AuNPs, we used bilayers with larger lipid patches and followed the fate of the lipid region immediately surrounding defects ( Fig. 5 ). After the addition of a different batch of 2:1 MUS:OT AuNPs (see Supplementary Fig. 7 for detailed chararacterization), light regions appear in the vicinity of the membrane edges in the AFM images. This change in topography is consistent with preferential particle insertion at the bilayer edge (c.f. Fig. 4 ). The protruding regions persist tens of nanometres away from the edges, suggesting that particles can extend their interaction away from the defect edge. The time evolution of these topography changes are shown in Supplementary Figs 8–10 . These results could be reproduced in a different SLB ( Supplementary Fig. 11 ). 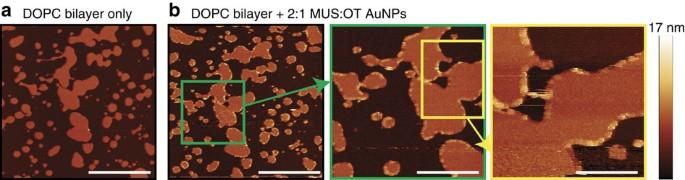Figure 5: Interactions of AuNPs with SLBs in the presence of large defects imaged by AFM. (a) Initial observation of lipid patches in the absence of added AuNPs. Scale bar, 2 μm. (b) The addition of 2:1 MUS:OT AuNPs to the solution leads to the formation of a higher area surrounding the defect edges as is clearly observed in the enlarged images. This change in topography is consistent with the insertion of AuNPs at bilayer edges and is observed in multiple bilayers (Supplementary Fig. 11). Scale bars, 2 μm and 800 and 400 nm from left to right. Figure 5: Interactions of AuNPs with SLBs in the presence of large defects imaged by AFM. ( a ) Initial observation of lipid patches in the absence of added AuNPs. Scale bar, 2 μm. ( b ) The addition of 2:1 MUS:OT AuNPs to the solution leads to the formation of a higher area surrounding the defect edges as is clearly observed in the enlarged images. This change in topography is consistent with the insertion of AuNPs at bilayer edges and is observed in multiple bilayers ( Supplementary Fig. 11 ). Scale bars, 2 μm and 800 and 400 nm from left to right. Full size image These experiments indicate that AuNPs do not insert into perfectly planar, defect-free SLBs, but are able to strongly attack the edges of large membrane defects. These findings are in strong agreement with the unbiased simulations that showed no membrane insertion through planar bilayers (akin to the defect-free SLBs) but showed immediate insertion through the highly curved ribbon edges (akin to the defect-rich SLBs). Moreover, the experiments indicate that this behaviour persists over timescales much longer than obtainable in simulations, and suggest that AuNPs can diffuse from the edge of defects into the bilayer bulk. Identification of transition state for insertion To understand why curvature mediates insertion, committor analysis was used with the atomistic simulations to identify the transition state for AuNP insertion [41] , [42] . For a system with two stable basins A and B in its free-energy landscape, the committor, p , is the probability that a trajectory initiated at a particular configuration will reach basin B before reaching basin A . The committor has a value of 0 for configurations in basin A and a value of 1 for configurations in basin B , with intermediate configurations lying in between these two extremes. If the committor is calculated for configurations lying on a transition path that connects these two basins, then the transition state can be identified as the configuration that has a value of p ≈0.5, where the system is equally likely to transition to either basin ( Supplementary Fig. 12 ). Committor analysis has been successfully used to identify the transition state in protein folding and vesicle fusion simulations similar to the system studied here [35] , [41] . p was calculated by extracting configurations from the two unbiased system trajectories in Fig. 3 . We associate basin A with a particle in solution and basin B with a particle inserted into the bilayer; because both basins are visited during these unbiased simulations, the trajectories are transition paths. A large series of independent simulations were launched from each of these extracted configurations after randomizing particle velocities, and p was calculated from the fraction that committed to basin B. Additional details are in the Supplementary Methods . 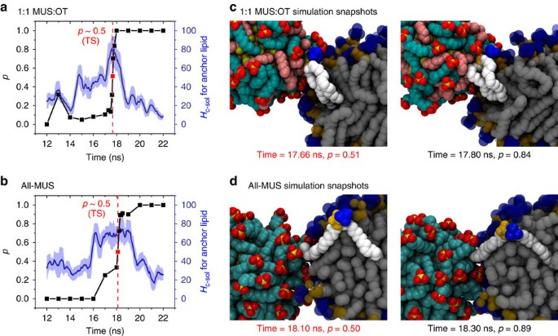Figure 6: Identification of the transition state (TS) for insertion. Plots of the committor,p, are shown as a function of time for insertion of the 1:1 MUS:OT (a) and all-MUS (b) particles. The committor obtains a value ofp≈0.5 at the TS, labelled in red. The number of hydrophobic contacts between solvent atoms and the single anchor lipid,Hc-sol, is shown in blue. The TS for both particles coincides with a maximum inHc-solwhere the anchor lipid can minimize water exposure by associating with either the bilayer or AuNP. Snapshots during and immediately after the TS are shown for both particles (c,d) with the anchor lipid emphasized to show the protrusion of an alkane tail through the solvated head group region of the bilayer and into contact with the AuNP. Some lipids are removed for clarity. Figure 6 shows the value of p as a function of the starting configuration time for both MUS:OT (a) and all-MUS (b) particles. The time axis corresponds to the same axis as in Fig. 3 constrained to the interval between 12 and 22 ns. The committor correctly goes from values near 0 for starting times corresponding to the initial surface fluctuation regime discussed previously to a value of 1 for times consistent with the insertion regime. The value of p ≈0.5 is found for a time t =17.66 ns for the 1:1 MUS:OT particle and t =18.10 ns for the all-MUS particle. The similarity in this transition time for both particles is likely coincidental. It must be emphasized that the value of the committor does not need to increase monotonically as a function of time for this unbiased trajectory. Figure 6a indeed shows that the committor increases at a time t =13 ns before decreasing and eventually increasing again as discussed in the Supplementary Methods . Figure 6: Identification of the transition state (TS) for insertion. Plots of the committor, p , are shown as a function of time for insertion of the 1:1 MUS:OT ( a ) and all-MUS ( b ) particles. The committor obtains a value of p ≈0.5 at the TS, labelled in red. The number of hydrophobic contacts between solvent atoms and the single anchor lipid, H c-sol , is shown in blue. The TS for both particles coincides with a maximum in H c-sol where the anchor lipid can minimize water exposure by associating with either the bilayer or AuNP. Snapshots during and immediately after the TS are shown for both particles ( c , d ) with the anchor lipid emphasized to show the protrusion of an alkane tail through the solvated head group region of the bilayer and into contact with the AuNP. Some lipids are removed for clarity. Full size image The key feature of the transition state is the protrusion of an aliphatic lipid tail into solvent and into contact with aliphatic groups in the AuNP monolayer. Analysis of the transition state for both trajectories revealed that only a single lipid tail was in contact with the AuNP surface in both cases (highlighted in Fig. 6 ). This ‘anchor’ lipid remained in contact for the duration of the simulation as the AuNP inserted into the bilayer ( Supplementary Fig. 13 ). For contact to occur between the anchor lipid and the AuNP, hydrophobic atoms in the lipid tail must first spontaneously fluctuate into the solvent region. Figure 6a,b shows the number of atoms in water molecules within 0.5 nm of any hydrophobic tail atoms in the anchor lipid, H c-sol , as a function of time, representing the amount of water unfavourably contacting the lipid of interest. Each point in Fig. 6 is averaged over ±100 ps to smooth fluctuations with the s.d. of this smoothing indicated by the transparent area. For both particles, the transition state coincides with a peak in H c-sol , which then decreases as p approaches 1. The broader transition for the committor for the all-MUS particle is similarly accompanied by a broader increase in H c-sol . These curves thus indicate that the transition state occurs when the anchor lipid is maximally exposed to water, a highly unfavourable state, and is close enough to contact the AuNP. To alleviate this solvent exposure, the lipid either relaxes back to the bulk of the bilayer or instead shields hydrophobic material within the AuNP monolayer, triggering bilayer insertion. The snapshots in Fig. 6c,d illustrate this process by highlighting the anchor lipid during and immediately following the transition state as it first protrudes into the solvated bilayer head region, increasing H c-sol , then preferentially increases contact with the particle. The recognition that insertion is initiated by the fluctuation of a lipid tail into solvent before contact with the AuNP explains why insertion is only observed at the highly curved bilayer edge in both simulations and experiments. At the bilayer edge, lipid tail protrusions into solvent are significantly enhanced in comparison with tail fluctuations in the middle of the bilayer ribbon, consistent with the higher average water contact shown in Fig. 2a and Supplementary Fig. 1 . AuNPs are thus more likely to contact a tail fluctuation that initiates insertion. This finding may imply that systems in which tail fluctuations are enhanced will generally reduce the kinetic barriers to insertion as discussed below. The prominent feature of the transition state identified in Fig. 6 is the protrusion of lipid tail into solvent before contact with the AuNP surface, a phenomenon extremely similar to the pre-stalk transition state proposed for vesicle–vesicle fusion [43] . Several recent simulation studies have shown that the pre-stalk transition for vesicle–vesicle fusion may involve the fluctuation of either a single lipid tail into solvent in a splayed configuration similar to the snapshots in Fig. 6d , or the fluctuation of two lipids from adjacent bilayers that make contact in the water layer between two vesicles in a configuration similar to the snapshots in Fig. 6c (refs 34 , 35 , 36 , 37 , 38 , 52 , 53 ). Several more examples of AuNP–lipid contacts are shown in Supplementary Fig. 14 and resemble these two states. Furthermore, previous simulations that did show vesicle–vesicle fusion did not observe fusion between vesicles and planar lipid bilayers [38] , [52] , similar to our observations of AuNP fusion with ribbon edges but not planar faces. Similarly, it has been shown previously both theoretically and experimentally that lipid tail protrusions and thus vesicle–vesicle fusion are enhanced for highly curved systems [38] , [54] , again agreeing with the results for the bilayer edge state presented here. Based on the findings from these vesicle studies and the current results, we conjecture that the same factors that enhance vesicle–vesicle fusion by stabilizing lipid fluctuations and the pre-fusion intermediate may also reduce the energy barrier for AuNP-bilayer fusion. Some examples of these factors are the presence of bilayer packing defects [55] , the lipid composition [56] and the generation of membrane stresses via transmembrane proteins [35] . While future work will be needed to establish that such factors affect AuNP insertion, there is some evidence in existing experimental results that supports the idea that enhanced lipid fluctuations reduce the barrier for AuNP insertion. In this study, hard substrates were used to support the planar lipid bilayers that may reduce lipid mobility by stabilizing the contacting lipid head groups [57] , [58] . This effect likely reduced the probability of tail protrusions, further limiting the insertion of AuNPs into the defect-free bilayers. In contrast, suspended lipid bilayers require less compressive force for fusion [59] and consequently measurements on suspended DOPC bilayers have indicated particle insertion [24] , [30] . While these suspended bilayers were also planar, the absence of a substrate allows for bilayer fluctuations, increasing the probability of lipid tail protrusions. Similarly, recent experimental work showed that AuNPs fused with lipid vesicles without allowing the passage of an impermeable membrane dye [25] . This can be explained by the increased probability of tail fluctuations with increasing vesicle curvature owing to larger amounts of exposed hydrophobic surface area [54] . The comparison between AuNP-bilayer fusion and vesicle–vesicle fusion is thus consistent with this study and previous experimental results, but future work will be necessary to fully establish that the kinetic barrier for AuNP insertion decreases in more fusogenic systems. The requirement of hydrophobic contact between both the lipid tails and hydrophobic material in the AuNP monolayer further suggests that monolayer properties should have a significant impact on the likelihood of insertion. The smaller number of successful insertions by all-MUS particles than MUS:OT particles observed in the simulations may be related to the lower probability that a lipid tail fluctuation contacts hydrophobic material in the all-MUS AuNP monolayer. It is likely that AuNP properties such as particle size, ligand composition and ligand length [44] also affect the probability of this hydrophobic contact. However, the key observation that lipid tail protrusions initiate insertion by contacting hydrophobic alkanethiol backbones for both all-MUS and MUS:OT AuNPs indicates that this behaviour may be general to a wide variety of monolayer compositions as this general chemical motif is prominent in a number of AuNP systems [9] , [10] , [31] , [60] , [61] , [62] . Moreover, the strong agreement with experimental results that used polydispserse particle batches with a larger mean core size than used in simulations implies that the pathway is similar for a range of particle core diameters. The identification of the transition state for insertion as coinciding with the first hydrophobic contact between the AuNP monolayer and lipid tails suggests that insertion is mediated by the hydrophobic effect, as would be expected based on previous free-energy calculations [25] , [32] . Supplementary Figure 15 shows that the hydrophobic solvent-accessible surface area (SASA) of the AuNP significantly decreases upon insertion that leads to a decrease in the free-energy penalty for hydrophobic solvation [63] . The SASA of the bilayer itself remains relatively unchanged during insertion, implying that it is AuNP properties that primarily drive insertion. The magnitude of the hydrophobic driving force is estimated from the SASA in the Supplementary Discussion and is similar to previous predictions from implicit models [25] , [32] , with upper bounds of −133.8 and −207.9 kcal mol −1 for the all-MUS and 1:1 MUS:OT particle, respectively. The stronger driving force for the more hydrophobic MUS:OT AuNPs may explain the greater magnitude of Δ x after 500 ns than the all-MUS particles ( Supplementary Fig. 3 ). The SLB experiments also suggest that AuNPs can diffuse into the middle of the bilayer ( Supplementary Fig. 10 ), far from the defect points. Such diffusion is not observed over the timescale of the simulations with Δ x reaching a plateau before 500 ns for both AuNP compositions. This plateau indicates that another energy barrier confines AuNPs near the defect edge and is likely related to the cost for lipid rearrangement when re-creating the bilayer edge. To determine whether there is a driving force for further insertion into the bilayer, we performed brief simulations with AuNPs fully embedded in the bilayer bulk. AuNPs were embedded in the bilayer by first creating a hole and then iteratively growing the AuNP into this void. Similar computational techniques are used to insert transmembrane proteins into bilayers [64] ( Supplementary Discussion ). A 2.0-nm all-MUS AuNP, 2.0-nm 1:1 MUS:OT AuNP and 3.0-nm 1:1 MUS:OT AuNP were all embedded using this method and the average SASA was measured to estimate the driving force for diffusion from the edge-inserted state to the centre of the bilayer. From these simulations, the driving force for further diffusion into the bilayer bulk was estimated as −22.1 kcal mol −1 for the 2.0-nm all-MUS AuNP and −107.7 kcal mol −1 for the 3.0-nm 1:1 MUS:OT AuNP. However, the SASA was unchanged upon further insertion of the 2.0-nm 1:1 MUS:OT AuNP. Inspection of the simulation snapshots at 500 ns ( Fig. 3 and Supplementary Fig. 4 ) indicates that unlike the all-MUS and larger MUS:OT AuNPs, the 2.0-nm MUS:OT AuNP has penetrated far enough into the bilayer that its edge has already been recreated. This particle has effectively penetrated into the bulk and further diffusion will likely occur but on a timescale longer than simulation times. Based on these considerations, we propose a pathway for edge-defect-mediated insertion of AuNPs into planar bilayers ( Fig. 7 ). Simulation snapshots of 2.0-nm all-MUS particles illustrate the variety of states through which the system transitions. First, the AuNP begins in solution (a) before electrostatic attraction drives the particle to the bilayer edge in a metastable state (b). The system then transitions through a first transition state associated with the fluctuations of lipid tails (TS 1), with the magnitude of the energy barrier related to the fusogenic properties of the bilayer. Driven by the hydrophobic effect, the particle then transitions to a metastable state inserted into the bilayer edge (c) where the hydrophobic SASA has decreased. A second barrier associated with the re-creation of the bilayer edge (TS 2) must then be crossed before the AuNP can attain a minimum free-energy state in the bulk of the bilayer (d). The magnitude of this barrier may also depend on AuNP properties; for example, the 2.0-nm 1:1 MUS:OT AuNP was observed to penetrate far enough into the bilayer that the edge reformed, implying a lower energy barrier for diffusion into the bulk as indicated by the dashed line in Fig. 7 . The magnitude of the overall free-energy change between states (a) and (d) was the subject of previous implicit models and depends on monolayer composition and particle size [25] , [32] . Having qualitatively identified the nature of these barriers, in future work we will compute quantitative values of these energy barriers using umbrella sampling techniques. Finally, while the experiments suggest that AuNPs insert at the defect edge then diffuse into the bulk as described in this pathway, it is also possible that previously embedded AuNPs may increase the probability of planar insertion in their vicinity by disrupting bilayer structure and enabling AuNPs to transition from states (a) to (d) directly. The effect of embedded AuNPs on bilayer structure will be the subject of future work to establish if such cooperative interactions occur. 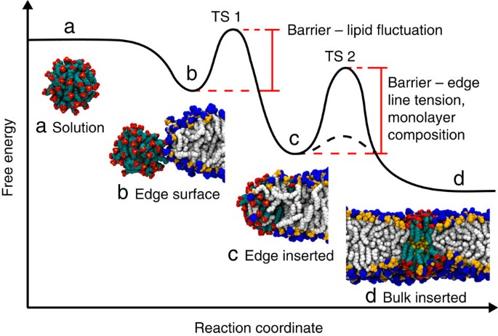Figure 7: Schematic of proposed pathway for defect-mediated bilayer insertion of AuNPs. From solution, the AuNP proceeds through multiple metastable points illustrated by the simulation snapshots. TS, transtion state. Figure 7: Schematic of proposed pathway for defect-mediated bilayer insertion of AuNPs. From solution, the AuNP proceeds through multiple metastable points illustrated by the simulation snapshots. TS, transtion state. Full size image To our knowledge, this is the first time that spontaneous membrane penetration by AuNPs has been observed in atomistic simulations that fully capture the structural, chemical and physical details of this complex bilayer-nanoparticle system. We expect that the physical insight gained from this study will be of great use in understanding AuNP-bilayer interactions. For example, the strong similarity of the AuNP-bilayer fusion process to the pre-stalk transition state for vesicle–vesicle fusion may allow these AuNPs to be used to probe the properties of fusogenic systems. Furthermore, the demonstration of strong thermodynamic forces associated with such insertion provides further evidence that such a process may explain recent experimental observations of non-disruptive association between AuNPs and bilayers [24] , [25] , [30] , [31] . Finally, the fusogenic properties of these AuNPs may present new opportunities for devising novel strategies for endosomal escape, drug delivery, controlled biodistribution and so on, all important research avenues for enhancing treatments based on nanomedicine. SLB preparation DOPC lipids in chloroform were purchased from Avanti Polar Lipids (Alabama, USA). The needed amount was put in a glass vial and the chloroform was let to evaporate overnight under vacuum. The PBS buffer, previously filtered with 200 nm singers’ filter, was added in the same vial to obtain a final concentration of 1 mg ml −1 DOPC in PBS. The 10 × PBS buffer (pH 7.4) was purchased from Ambion and diluted 10 × with Milli-Q water (18.2 MΩ, <4 p.p.m. organics; Merck-Milipore, Billerica, MA, USA). The 1 mg ml −1 DOPC solution in PBS was sonicated for 10 min and vortexed. Successively, 1 ml of 1 mg ml −1 DOPC in PBS was extruded 21 times at room temperature through a membrane with 100 nm pores (PC Membranes 0.1 μm, Avanti Polar Lipids). The solution obtained was successively diluted 10 times, obtaining a final concentration of 0.1 mg ml −1 of DOPC vesicles in PBS. This solution was used in both AFM and QCM-D experiments. The silicon oxide substrates were obtained from p-doped silicon wafers. Substrates with the desired dimensions were cut with a diamond tip and successively cleaned as described in the Supplementary Methods . The SLBs for the AFM experiments on silicon wafer were obtained via vesicle deposition. A drop of 0.1 mg ml −1 solution of DOPC vesicles in PBS was put on top of the substrates and the system was heated to 40 °C for 20–30 min. Extra PBS buffer was added and the substrates were rinsed copiously with the pipette tips making sure that no air bubbles made contact with the surface. The PBS was successively exchanged at least three times before transferring the substrates to the Teflon Petri dish for the AFM measurement. AuNP synthesis All chemicals were purchased from Sigma-Aldrich except for the ligand MUS, which was synthesized following the procedure of Verma et al . [26] All solvents purchased were reagent grade and purged with nitrogen gas for >30 min before the reaction. All particles were synthesized following a modification on the procedure reported by Zheng et al . [65] The solvent used was a 10% Milli-Q water in dimethylformamide mixture. The targeted amounts of chloro(triphenylphosphine)gold(I) (Sigma), MUS plus OT ligands, and the reducing agent borane tert-butylamine (Sigma) complex were measured and dissolved separately by sonication in 20 ml glass vials. The gold salt solution was added to ≈100 ml of the solvent mixture at room temperature in a 250-ml round bottom flask under magnetic stirring (≈800 r.p.m. ), followed by the addition of the thiol mixture. After 10 min, the solution became turbid and the reducing agent solution was added. The flask was capped with a condenser and brought to reflux between 120 and 125 °C. The reaction was stirred for 1.5 h then the heat was turned off and the solution was cooled at room temperature, under stirring, for another 1.5 h. The flask was placed in a 4 °C fridge overnight, after which the product precipitated and the supernatant was discarded. The product was washed several times (3–5) by suspending and centrifuging (5,500 r.p.m.) it in acetone then ethanol. Finally, the product was washed five times with Milli-Q water using Amicon Ultra-15 centrifugal filter devices, 10 kDa NMWL (Nominal Molecular Weight Limit). Amplitude modulation-AFM imaging in liquid All the AFM measurements were carried out in liquid with a commercial MFP-3D AFM (Asylum Research, Santa Barbara, CA, USA). We used a triangular silicon nitride cantilever (TR400-PSA, Olympus, Japan) with a nominal stiffness of k =0.23 N m −1 or a rectangular silicon nitride cantilever (RC800-PSA, Olympus) with a nominal stiffness of k =0.05 N m -1 . The cantilevers were fully immersed in the liquid for the experiment. The samples were mounted on a homemade Teflon Petri dish and fixed mechanically using a Teflon O-ring. After the transfer of the samples to the Petri dishes the PBS solution was exchanged several times and finally mounted with standard magnetic supports on the AFM stage. The transfer procedure of the substrates from the PBS solution to the AFM stage was carried out with extreme caution to make sure that the lipid bilayers obtained on the silicon wafers were never in contact with air or air bubbles, compromising their integrity. If required, we intentionally dewetted the lipid bilayer to create defects. The system was then allowed to thermalize at room temperature (24 °C) for 30–60 min in order to minimize drift before acquiring data. The AFM was operated in amplitude-modulation mode (‘tapping’ in the AFM commercial software) with the setpoint/free amplitude ratio ( A/A 0 ) as high as possible (typically A/A 0 >0.8). The samples were imaged in standard PBS. If the surface did not show signs of any defects, such as holes with specific height values (4–5 nm) that is a clear signature of the presence of DOPC bilayers, a series of force curves were performed to test the presence of the bilayers. Successively the tip was withdrawn from the surface and 100 μl of 10 mg ml −1 AuNPs solution was added. Immediately afterwards, contact with the surface was again established and we followed the change in time of the surface topography. Image analysis was performed using SPIP (Image Metrology, Denmark), Gwyddion ( http://gwyddion.net ) and Igor Pro (Wavemetrics, Lake Oswego, OR, USA). The images were flattened and eventually low-pass filtered to remove high frequency noise. QCM-D experiments All the QCM-D measurements were carried out with the commercial QCM-D machine Q-Sense E4 (Biolin Scientific/Q-Sense, Västra Frölunda, Sweden) connecting the four sensors to a standard Ismatec IPC-N 4 peristaltic pump (IDEX Health & Science GmbH, Wertheim, Germany). The four silicon oxide sensors were ordered directly from Q-sense. Before the beginning of the experiments the sensors were placed in the chambers, sealed and heated to 40 °C. The QCM-D experiments were performed at this temperature to help the formation of the DOPC bilayer during the initial stage of the experiment. This temperature was maintained during all experiments using the temperature control system of the machine. We prepared glass vials, previously cleaned, filled with Milli-Q water, PBS, AuNPs solution and 0.1 mg ml −1 of DOPC vesicles (100 nm in diameter) in PBS. All the solvents, excluding the vesicles in PBS, were sonicated before use to degas them and limit the formation of air bubbles during the experiment. The solutions were put in a water bath at 45 °C during the experiments and before insertion into the tubing system to avoid the formation of air bubbles in the Teflon tubes and in the QCM chambers. The flux velocity used in all experiments was of 100 μl min −1 unless the presence of an air bubble was detected. The first step in the actual experiment was to flush using only PBS for at least 30 min, allowing the system to equilibrate. The standard value of frequency drift obtained was of <1 Hz min −1 . Subsequently the suspension of lipid vesicles in PBS was injected and the signal of bilayer formation was recorded. After 10 min, new PBS solution was injected to remove any extra unfused vesicles in solution. At this stage the system was left to equilibrate for 30 min. Occasionally, the first overtone showed the signature of the presence of air bubbles that were removed by flushing PBS at maximum speed in both directions. Successively, the AuNP suspension (concentration of 1 mg ml −1 ) was injected in the QCM chambers for several minutes. Finally, new clean PBS was inserted into the tubing system to exclude the effect of the solvent change in the recorded signal and have a clean reference. Simulation methods The DOPC bilayer, water, ions and AuNPs were all modelled with the GROMOS 54a7 force field [44] , [46] , [47] . Some modifications were made to incorporate gold ( Supplementary Methods ). In binary monolayers, the MUS and OT ligands segregate into a stripe-like morphology that may have a role in cellular penetration [8] , [26] , [27] . However, in our previous work, we found no distinction between a stripe-like morphology and a more uniform ‘checkerboard’ arrangement of ligands on the thermodynamics of insertion in model bilayers [25] , [32] . Therefore, the simulations here use the uniform ‘checkerboard’ arrangement of ligands in the 1:1 MUS:OT monolayers to approximate an isotropic ligand distribution [44] . For all simulations, bond lengths were constrained using the LINCS algorithm [66] . The simple point charge water model with the water geometry constrained using the SETTLE algorithm [67] . The simulation timestep was set to 2 fs for the molecular dynamics integrator. Electrostatic interactions were calculated using the particle-mesh Ewald summation method (PME) with a real-space cutoff of 1.0 nm, a grid spacing of 0.12 nm and fourth-order interpolation [47] . The van der Waals and neighbour list cutoffs were also both set to 1.0 nm in accordance with recent simulations of lipid bilayers using PME and the GROMOS 54a7 parameter set [47] . The temperature of the system was set to 37 °C using a velocity rescale thermostat with a time constant of 0.1 ps. The pressure was fixed at 1 bar using an anisotropic Berendsen barostat with a time constant of 5.0 ps. The reference pressure and compressibility were set to 0 in the y dimension to eliminate box motion while allowing box motion in the x / z dimensions with a reference pressure of 1 bar and a compressibility of 4.5 × 10 −5 bar −1 . This barostat scheme was used to preserve the ribbon geometry described below. All simulations were run with the Gromacs package version 4.6.1 (ref. 68 ). The DOPC bilayer was assembled as a ribbon following the protocol described recently by West et al . [69] The ribbon was constructed by first equilibrating a 200 lipid bilayer at constant volume and pressure for 100 ns, then duplicating the bilayer in the x direction while adding additional water to put 10 nm of space between the edges of the 400 lipid bilayer across the periodic boundaries before re-equilibrating. Committor analysis The committor was calculated by first extracting a series of starting configurations in 1 ns intervals between the 12 and 22 ns time points for both trajectories shown in Fig. 3 . In addition, more fine-grained starting points were then extracted after initial analysis to more accurately locate the transition state. For each starting configuration, 20 simulations were run for 2 ns each after first randomizing the starting velocities of all particles. This short time was possible because of the rapid decrease in Δ x that marks initial commitment to insertion. The length of the short trajectories should be on the order of the commitment time [42] , so 2 ns was sufficient to gauge commitment and also permitted large numbers of simulations to be run. An additional 20 simulations were run if 0.05< p <0.95 after the initial 20 simulations to improve sampling. Simulations were characterized as committed to basin A or B as judged by two order parameters: the previously defined distance Δ x and the number of hydrophobic contacts, H c , between lipid tail atoms and hydrophobic atoms in the ligand monolayer. A hydrophobic contact was counted if two atoms were within 0.5 nm of each other. These parameters were selected on the basis of observations during the unbiased trajectories. A trajectory was marked as committed to B if Δ x <−1.0 nm and if H c >50 at the end of the run trajectory. A trajectory was marked as committed to A if Δ x >−0.5 nm or if H c <5. Finally, simulations that did not meet either criteria at the end of the run were marked as uncommitted and did not contribute to the calculation of p . This typically occurred when the distance had decreased below the threshold but the number of hydrophobic contacts, while possibly >0, was still less than the threshold and fluctuated during the trajectory. How to cite this article: Van Lehn, R. C. et al. Lipid tail protrusions mediate the insertion of nanoparticles into model cell membranes. Nat. Commun. 5:4482 doi: 10.1038/ncomms5482 (2014).